AirwayPrevotellapromote TLR2-dependent neutrophil activation and rapid clearance ofStreptococcus pneumoniaefrom the lung 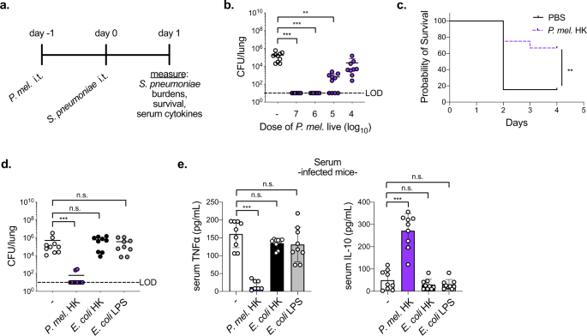Fig. 1: Exposure to airwayP. melaninogenica(P. mel.) induces rapid clearance ofS. pneumoniae. aTimeline forPrevotellaexposure followed byS. pneumoniaeinfection.bLung type 2S. pneumoniaeburdens following exposure to PBS (-) or liveP. mel. strain 25845 i.t. at indicated doses prior to 24 h infection withS. pneumoniae, 5×106CFU/mouse (n= 10 mice/group).cSurvival following exposure to PBS orP. mel. heat-killed (HK, 107CFU equivalents/mouse) i.t. prior toS. pneumoniaeinfection, 107CFU/mouse (n= 13 mice/group).d,eLungS. pneumoniaeburdens (d) and serum cytokines (e) in mice following exposure to PBS (-),P. mel. HK,E. coliHK, orE. colilipopolysaccharide (LPS) i.t. prior to 24 hS. pneumoniaeinfection, 5×106CFU/mouse (n= 10 mice/group). LOD = limit of detection. Data are pooled from three independent experiments, displayed as mean ± SEM. Forbfrom left to right ***p< 0.0001, ***p< 0.0001, **p= 0.0015, Kruskal–Wallis with Dunn’s post hoc test,c**p= 0.0075, Mantel-Cox survival test,dfrom left to right ***p= 0.0008,p> 0.9999,p> 0.9999, Kruskal–Wallis with Dunn’s post hoc test,efrom left to right ***p< 0.0001,p= 0.2352,p= 0.1558 (TNFα), from left to right ***p< 0.0001,p= 0.6977,p= 0.7136 (IL-10), one-way ANOVA with Dunnett’s post hoc test. Source data are provided as a Source Data file. This study investigates how specific members of the lung microbiome influence the early immune response to infection. Prevotella species are a major component of the endogenous airway microbiota. Increased abundance of Prevotella melaninogenica correlates with reduced infection with the bacterial pathogen Streptococcus pneumoniae , indicating a potentially beneficial role. Here, we show that P. melaninogenica enhances protection against S. pneumoniae , resulting in rapid pathogen clearance from the lung and improved survival in a mouse lung co-infection model. This response requires recognition of P. melaninogenica lipoproteins by toll-like receptor (TLR)2, the induction of TNFα, and neutrophils, as the loss of any of these factors abrogates Prevotella -induced protection. Improved clearance of S. pneumoniae is associated with increased serine protease-mediated killing by lung neutrophils and restraint of P. melaninogenica -induced inflammation by IL-10 in co-infected mice. Together, these findings highlight innate immune priming by airway Prevotella as an important protective feature in the respiratory tract. The respiratory tract is home to a diverse microbial community that varies in composition by anatomical location and over the course of life. Prevotella are frequently identified as one of the top three most abundant bacteria detected in the oral cavity and lungs of healthy adults [1] , [2] , [3] , [4] . While the largest biomass and most stable microbial communities in the respiratory tract are located in the upper airway, the lung is constantly exposed to these bacteria by micro-aspiration. Bacteria from the oral cavity are the dominant source of lung microbiome “seeding” [1] , [2] . In the absence of the steep oxygen gradients that arise during chronic lung infection, sustained growth of obligate anaerobes such as Prevotella in the lung remains debated, but frequent exposures may nevertheless function as an important immune regulatory signal. The purpose of this study was to determine how airway Prevotella influence the early immune response to infection with the bacterial pathogen Streptococcus pneumoniae (the pneumococcus). S. pneumoniae is the most common cause of community-acquired pneumonia, which has an estimated economic impact of $17 billion in the U.S. alone and is the leading cause of death in children under 5 years old [5] , [6] . Pneumococcal vaccines are extremely effective against invasive disease, but are not as protective against pneumonia, and the phenomenon of serotype replacement has increased the number of non-vaccine strains in circulation [7] . Asymptomatic colonization of the nasopharynx with S. pneumoniae is a prerequisite for disease development, following invasion to other tissues including the lung. However, it remains unclear why some individuals are more predisposed to lung infection with S. pneumoniae compared with others. The microbiome is thought to help protect against bacterial lung infections, which are worsened in antibiotic treated and germ-free mice [8] , [9] . S. pneumoniae also persists more readily following antibiotic therapy [10] . Prevotella are a candidate “protective” member of the airway microbiome in the context of S. pneumoniae infection, as several studies indicate an association between increased abundance of Prevotella and reduced S. pneumoniae in both the upper airway [11] , [12] and lung [2] , [13] , [14] . Similarly, Prevotella species including P. melaninogenica are more abundant in healthy adults than those with pneumonia [15] , [16] . While species-level classification in such analyses is limited, in one report P. melaninogenica was ranked as the most discriminative operational taxonomic unit (OTU) differentiating healthy adults from patients with pneumococcal pneumonia [12] . P. melaninogenica is an important member of the endogenous airway microbiota, as it is part of the core oral microbiome [17] , [18] and selectively enriched in the lung [1] , [4] , [19] . The factors underlying the potential benefit of airway Prevotella on protection against pneumococcal pneumonia are unresolved. In healthy adults, the enrichment of Prevotella rRNA gene concentration in bronchoalveolar lavage fluid (BAL) is associated with sub-clinical inflammation, including increased numbers of activated neutrophils [20] . However, Prevotella -induced inflammation is subdued compared to that induced by opportunistic bacterial pathogens. For example, lung transplant recipients with Prevotella -dominant BAL microbiome profiles had lower innate immune activation profiles than those with Staphylococcus or Pseudomonas -dominant microbiomes [21] . In mice, lung exposure to Prevotella melaninogenica induced less toll-like receptor(TLR)2-dependent inflammation than the pathogen Haemophilus influenzae [22] . Similarly, another Prevotella species induced TLR2 signaling but fewer pro-inflammatory cytokines than a cystic fibrosis (CF) pathogen in human CF bronchial epithelial cells [23] . In the context of CF, both positive and negative roles have been attributed to anaerobic bacteria including P. melaninogenica , though Prevotella abundance correlates with milder CF in some cases [24] . Prevotella species are not universally beneficial or benign members of the airway microbiome. Unlike P. melaninogenica , Prevotella intermedia is frequently isolated from periodontal abscesses, expresses virulence factors including a type 6 secretion system (T6SS), and enhances susceptibility to S. pneumoniae by upregulating a critical host adherence receptor [25] , [26] . P. melaninogenica has been identified in polymicrobial lung abscesses, though it is unclear which species drive abscess formation, and causes increased tissue damage in the context of bleomycin-induced pulmonary fibrosis in mice [27] . These studies suggest that the overall beneficial versus detrimental effects of Prevotella on airway health depend on the amplitude and context of Prevotella -induced immune responses. For this study, we developed an animal model to determine how airway Prevotell a modulate innate immune-mediated protection against S. pneumoniae . Using this model, we identify an innate immune response induced by several Prevotella species including P. melaninogenica associated with rapid clearance of S. pneumoniae from the lung, highlighting airway Prevotella as an important immune regulatory signature that contributes to respiratory tract health. P. melaninogenica enhances clearance of S. pneumoniae While the murine airway microbiome contains both Prevotella and Streptococcus species, the strains used in these studies are not resident members, allowing us to control exposures to each bacterium. Prevotella aspiration was modeled in mice by instilling P. melaninogenica intratracheally (i.t.) prior to challenge with S. pneumoniae (Fig. 1a ). S. pneumoniae burdens at 24 h post-infection were not detected in any mice pre-exposed to an equivalent dose of live P. melaninogenica , compared to burdens of ~10 5 colony forming units (CFUs) in mice infected with S. pneumoniae alone (Fig. 1b ). Titration of P. melaninogenica revealed that significant protection was maintained with up to a 100-fold lower dose of live P. melaninogenica than that of S. pneumoniae (Fig. 1b ). Burdens of 10 5 CFU/mL P. melaninogenica have been reported in human lung lavage fluid [19] , which falls within this protective range. These data suggest that exposure to live P. melaninogenica mediates rapid clearance of S. pneumoniae from the murine lung. Fig. 1: Exposure to airway P. melaninogenica ( P. mel .) induces rapid clearance of S. pneumoniae . a Timeline for Prevotella exposure followed by S. pneumoniae infection. b Lung type 2 S. pneumoniae burdens following exposure to PBS (-) or live P. mel . strain 25845 i.t. at indicated doses prior to 24 h infection with S. pneumoniae , 5×10 6 CFU/mouse ( n = 10 mice/group). c Survival following exposure to PBS or P. mel . heat-killed (HK, 10 7 CFU equivalents/mouse) i.t. prior to S. pneumoniae infection, 10 7 CFU/mouse ( n = 13 mice/group). d , e Lung S. pneumoniae burdens ( d ) and serum cytokines ( e ) in mice following exposure to PBS (-), P. mel . HK, E. coli HK, or E. coli lipopolysaccharide (LPS) i.t. prior to 24 h S. pneumoniae infection, 5×10 6 CFU/mouse ( n = 10 mice/group). LOD = limit of detection. Data are pooled from three independent experiments, displayed as mean ± SEM. For b from left to right *** p < 0.0001, *** p < 0.0001, ** p = 0.0015, Kruskal–Wallis with Dunn’s post hoc test, c ** p = 0.0075, Mantel-Cox survival test, d from left to right *** p = 0.0008, p > 0.9999, p > 0.9999, Kruskal–Wallis with Dunn’s post hoc test, e from left to right *** p < 0.0001, p = 0.2352, p = 0.1558 (TNFα), from left to right *** p < 0.0001, p = 0.6977, p = 0.7136 (IL-10), one-way ANOVA with Dunnett’s post hoc test. Source data are provided as a Source Data file. Full size image We next examined the impact of inactivated (heat-killed, HK) P. melaninogenica on survival following a lethal dose of S. pneumoniae . Exposure to P. melaninogenica significantly increased the probability of survival, with 33% of Prevotella -exposed mice succumbing to infection compared to 85% of mice infected with S. pneumoniae alone (Fig. 1c ). Improved survival in mice exposed to P. melaninogenica correlated with lower pneumococcal burdens in the lung 3 days post-infection (Supplementary Fig. 1a ). The rapid protection induced by P. melaninogenica was not dependent on instillation of Prevotella into the lung, as intranasal inoculation similarly enhanced S. pneumoniae clearance by 24 h (Supplementary Fig. 1b ). P. melaninogenica was protective against both serotype 2 S. pneumoniae , which spreads systemically by 24 h, and serotype 3 S. pneumoniae , which is restricted to the lung (Fig. 1c, d ). Together, these data indicate that exposure to live or inactivated P. melaninogenica protects against S. pneumoniae infection. We next determined whether instillation of any HK bacterium enhances protection against S. pneumoniae . Initially, we investigated other HK bacteria which are common members of the upper airway microbiota and are known to mediate direct competition with S. pneumoniae , including two Corynebacterium species [28] , [29] and Streptococcus salivarius [30] . In contrast to live strains, two of which reduce S. pneumoniae infection in a similar pre-exposure model [29] , none of the HK strains were protective (Supplementary Fig. 1e ), indicating a unique effect mediated by P. melaninogenica HK compared with these airway commensals, which like S. pneumoniae are Gram-positive. P. melaninogenica is a Gram-negative bacterium, and the lipopolysaccharide (LPS) of Gram-negative bacteria is an abundant TLR4 agonist. We next compared the impact of exposure to Gram-negative Escherichia coli HK as well as E. coli LPS, which improves protection against other lung pathogens by immune priming [31] , [32] . Unlike P. melaninogenica , neither E. coli HK nor E. coli LPS enhanced clearance of S. pneumoniae from the lung (Fig. 1d ), suggesting that not all Gram-negative bacteria have a similar effect. Systemic cytokine responses also differed in mice exposed to P. melaninogenica compared with E. coli HK or E. coli LPS (Fig. 1e ). These findings indicate that P. melaninogenica , but not E. coli LPS, enhances protection against S. pneumoniae lung infection, allowing for the use of E. coli LPS as an immune stimulatory but non-protective comparative tool. P. melaninogenica activates lung neutrophils The rapid protective effect of P. melaninogenica implies a role for the innate immune system. We focused on the use of P. melaninogenica HK to investigate the mechanism of this effect, as burdens of live P. melaninogenica may themselves be altered by the disruption of innate immune pathways. The immune response induced by P. melaninogenica HK was first examined in the absence of S. pneumoniae infection. P. melaninogenica exposure increased the production of several pro-inflammatory cytokines in lung bronchoalveolar lavage fluid (BAL), including TNFα, IL-6, IL-1α, and IFNγ as well as the chemokines MCP-1 (CCL2) and MIP-2 (CXCL2), a major neutrophil chemoattractant [33] (Fig. 2a ). P. melaninogenica also increased systemic TNFα and IL-10 compared to mice treated with PBS or E. coli LPS (Fig. 2b ). The recruitment and activation of innate immune cells in the lung was evaluated by intracellular flow cytometry (Supplementary Fig. 2a ). P. melaninogenica significantly enhanced the recruitment of myeloid cells including inflammatory monocytes and neutrophils, similar to E. coli LPS (Fig. 2c, d and Supplementary Fig. 2b, c ). However, unlike E. coli LPS, P. melaninogenica also induced TNFα production in lung neutrophils (Fig. 2e ). Neither stimulus affected the recruitment or TNFα production of CD11b hi dendritic cells (DCs) (Supplementary Fig. 2d, e ). These data indicate that exposure to P. melaninogenica induces a pro-inflammatory response in the lung associated with increased neutrophil recruitment and activation. Fig. 2: P. melaninogenica ( P. mel.) induces a pro-inflammatory immune response in the lung associated with neutrophil activation in the absence of S. pneumoniae infection. a Quantification of cytokines and chemokines in lung bronchoalveolar lavage (BAL) following exposure to PBS (-) or P. mel . heat-killed (HK) strain 25845 i.t. for 24 h ( n = 10 mice/group). b Serum cytokines detected in mice exposed to PBS (-), P. mel . HK, or E. coli lipopolysaccharide (LPS) i.t. for 24 h ( n = 5 mice/group). c – e Percentage and total number of inflammatory monocytes (CD45 + SiglecF - Ly6G - Ly6C + CD11b + cells) ( c ), neutrophils (CD45 + SiglecF - Ly6G + CD11b + cells) ( d ), and neutrophil TNFα ( e ) detected in the lungs of mice from b by intracellular flow cytometry, with representative plots shown for the percentage of neutrophils and neutrophil TNFα ( n = 5 mice/group). Data are pooled from three independent experiments ( a ) or representative from one of four independent experiments ( b – e ). Box boundaries in a indicate the 25th and 75th percentiles, with a horizontal line representing the median and whiskers indicating minimum and maximum values. Data in b – e are displayed as mean ± SEM. For a *** p < 0.0001, two-way ANOVA with Sidak’s post hoc test, b from left to right *** p < 0.0001, p = 0.9108 (TNFα), *** p < 0.0001, p = 0.9108 (IL-10), one-way ANOVA with Dunnett’s post hoc test and from left to right p = 0.0060, p > 0.9999 (TNFα), p = 0.0144, p > 0.9999 (IL-10), Kruskal–Wallis with Dunn’s post hoc test, c from left to right ** p = 0.0044, * p = 0.0453, p = 0.9875, p = 0.5395, Kruskal–Wallis with Dunn’s post hoc test, d from left to right *** p = 0.009, ** p = 0.0017, one-way ANOVA with Dunnett’s post hoc test and p = 0.0115, p = 0.0215, Kruskal–Wallis with Dunn’s post hoc test, e from left to right *** p < 0.0001, p = 0.7296, one-way ANOVA with Dunnett’s post hoc test and p = 0.0008, p = 0.1542, Kruskal–Wallis with Dunn’s post hoc test. Source data are p rovided as a Source Data file. Full size image P. melaninogenica- exposed mice had fewer alveolar macrophages (AMs) in their lungs than mice exposed to either PBS or E. coli LPS (Supplementary Fig. 2f ). Others have reported that E. coli LPS activates AM production of TNFα, which we confirm, though this response was not induced by P. melaninogenica (Supplementary Fig. 2g ). These findings indicate distinct lung innate immune cell activation profiles for mice exposed to E. coli LPS compared with P. melaninogenica , which unlike E. coli LPS is protective against S. pneumoniae . Neutrophils and TNFα are critical for P. melaninogenica protection Neutrophils are important for S. pneumoniae killing at early time points, prior to the development of specific immunity, which is typically required for clearance [34] . Exposure to P. melaninogenica HK increased the number of neutrophils recruited to the lungs in response to S. pneumoniae infection (Fig. 3a ). To address the contribution of neutrophils to pneumococcal clearance in Prevotella -exposed mice, we depleted neutrophils prior to S. pneumoniae infection. In the absence of neutrophils, P. melaninogenica was no longer protective against S. pneumoniae , as lung burdens in Prevotella -exposed mice were similar to those in mice infected with S. pneumoniae alone (Fig. 3b ). These data indicate that neutrophils are required for P. melaninogenica -mediated protection against S. pneumoniae . Fig. 3: Neutrophils and TNFα are critical for P. melaninogenica ( P. mel . )-mediated protection against S. pneumoniae infection. a , b Representative flow cytometry plots and total cell numbers for neutrophils detected by flow cytometry ( n = 5 mice/group, PBS, n = 4 mice/group, others) ( a ) and lung burdens of type 2 S. pneumoniae ( n = 9 mice/group) ( b ) in mice treated with isotype control or anti-Ly6G antibodies (200 μg/mouse) i.p. together with either PBS (-) or P. mel . strain 25845 heat-killed (HK) i.t. prior to 24 h S. pneumoniae infection, 5×10 6 CFU/mouse. c – e Total cell number of neutrophils and neutrophil TNFα detected by intracellular flow cytometry ( n = 5 mice/group for isotype control groups, 4 mice/group for anti-TNFα groups) ( c , d ) and lung S. pneumoniae burdens ( n = 9 mice/group) ( e ) in mice treated with isotype control or anti-TNFα antibodies (200 μg/mouse) i.p. together with either PBS (-) or P. mel . HK i.t. prior to 24 h S. pneumoniae infection. LOD = limit of detection. Data are pooled from three independent experiments ( b , e ) or representative from one of four independent experiments ( a , c , d ), displayed as mean ± SEM. For a * **p < 0.0001, one-way ANOVA with Sidak’s post hoc test, b from left to right * p = 0.0222, p > 0.9999, p = 0.0751, * p = 0.0192, Kruskal–Wallis with Dunn’s post hoc test, c from left to right * p = 0.0337, *** p < 0.0001 one-way ANOVA with Tukey’s post hoc test, d ** p = 0.003, *** p = 0.0002 one-way ANOVA with Tukey’s post hoc test, e from left to right p = 0.3058, p > 0.9999, p = 0.4470, * p = 0.0118, Kruskal–Wallis with Dunn’s post hoc test. Source data are provided as a Source Data file. Full size image P. melaninogenica -induced TNFα was significantly reduced in the lungs of neutrophil-depleted mice, indicating neutrophils as a major source of TNFα in this setting (Supplementary Fig. 2h ). We next considered whether the pro-inflammatory response associated with elevated neutrophil TNFα is required for P. melaninogenica -mediated protection by depleting TNFα. Neutrophil recruitment and production of TNFα were reduced in TNFα-depleted mice (Fig. 3c, d , and Supplementary Fig. 3a, b ). Similar to the effect of neutrophil depletion, TNFα depletion resulted in loss of P. melaninogenica- mediated protection (Fig. 3e ). Inflammatory monocyte recruitment was also reduced in TNFα depleted mice, though CD11b hi DCs and AM populations were unchanged (Supplementary Fig. 3c–e ). Together, these data indicate a requirement for both neutrophils and TNFα in P. melaninogenica- mediated protection against S. pneumoniae . P. melaninogenica is protective in microbiome-depleted mice While our findings suggest that innate immune priming is important for P. melaninogenica -mediated protection, it was unclear whether the endogenous microbiome, which regulates immune homeostasis, is required for this protective effect. The contribution of the endogenous microbiome to protection in Prevotella -exposed mice was evaluated using antibiotic treated and Germ-free mice. In antibiotic treated mice, live P. melaninogenica significantly improved S. pneumoniae clearance from the lungs by 24 h (Fig. 4a and Supplementary Fig. 4a ). Similarly, exposure to live P. melaninogenica enhanced clearance of S. pneumoniae from the lungs of Germ-free mice (Fig. 4b ). In Germ-free mice, Prevotella -mediated protection against S. pneumoniae was associated with increased lung neutrophil recruitment and activation (Fig. 4c and Supplementary Fig. 4b ). These data indicate that P. melaninogenica is sufficient to improve protection against S. pneumoniae lung infection in the absence of an intact microbiome. Fig. 4: P. melaninogenica ( P. mel .) is protective against S. pneumoniae infection in microbiome-depleted mice. a Lung S. pneumoniae burdens in mice treated with antibiotics followed by exposure to PBS (-) or live P. mel . strain 25845 i.t. prior to 24 h S. pneumoniae infection, 5 × 10 6 CFU/mouse ( n = 9 mice/group). b , c Lung S. pneumoniae burdens ( b ) and percent neutrophils, neutrophil TNFα ( c ) in Germ-free mice treated with either PBS (-) or live P. mel . i.t. prior to 24 h S. pneumoniae infection, 10 6 CFU/mouse ( n = 11 mice/group). LOD = limit of detection. Data are pooled from three independent experiments. Data are displayed as mean ± SEM. For a , b *** p < 0.0001 two-tailed Mann–Whitney U -test, c *** p < 0.0001 two-tailed t -test. Source data are provided as a Source Data file. Full size image P. melaninogenica lipoproteins induce TLR2-dependent neutrophil TNFα We next investigated the host and bacterial requirements for P. melaninogenica -induced neutrophil TNFα in vitro. In neutrophils purified from the bone marrow of naïve mice, exposure to P. melaninogenica HK induced TNFα secretion in a dose-dependent manner (Fig. 5a ). Small molecule inhibitors of TLR2 (C29) [35] and TLR4 (TAK-242) [36] were used to compare the importance of TLR2 versus TLR4 for P. melaninogenica- induced TNFα. Inhibition of TLR2, but not TLR4, resulted in loss of P. melaninogenica -induced neutrophil TNFα (Fig. 5b ), suggesting that TLR2 signaling is important for this response. In support of this conclusion, P. melaninogenica- induced TNFα secretion was absent in neutrophils purified from TLR2 deficient ( Tlr2 −/− ) mice, in contrast to neutrophils from wild-type (WT) mice (Fig. 5c ). These data indicate that TLR2 is required for P. melaninogenica stimulation of neutrophil TNFα secretion. Fig. 5: P. melaninogenica ( P. mel .) lipoproteins induce neutrophil TNFα secretion in a TLR2-dependent manner. a Supernatant TNFα detected 24 h following incubation of bone marrow (BM) neutrophils purified from naïve wild-type (WT) mice with P. mel . strain 25845 heat-killed (HK) at the indicated ratios ( n = 3 independent experiments/group). b Supernatant TNFα detected 24 h following incubation of BM neutrophils from WT mice incubated with P. mel . HK (1:1 ratio) with and without inhibitors of TLR2 (C29) or TLR4 (TAK-242), ( n = 3 independent experiments/group). c Supernatant TNFα detected 24 h following incubation of BM neutrophils from WT or Tlr2 -/- mice with PBS (-), P. mel . HK (1:1 ratio), P. mel . lipopolysaccharide (LPS, 10 ng/mL), P. mel . lipoproteins (10 ng/mL), or Pam3SK4 (10 ng/mL), ( n = 3 independent experiments/group). d Supernatant TNFα detected 24 h following incubation of BM neutrophils from WT mice treated with PBS (-), untreated P. mel . HK, or lipoprotein-digested P. mel . HK ( n = 3 independent experiments/group). e Lung type 2 S. pneumoniae burdens in mice treated with PBS (-), untreated P. mel . HK, or lipoprotein-digested P. mel . HK i.t. prior to 24 h S. pneumoniae infection, 5×10 6 CFU/mouse ( n = 9 mice/group). f Lung S. pneumoniae burdens in mice treated with PBS (-, n = 11 mice), P. mel . lipoproteins (10 μg/mouse, n = 9 mice), or Pam3SK4 (10 μg/mouse, n = 10 mice, 25 μg/mouse, n = 8 mice, or 50 μg/mouse, n = 8 mice) i.t. prior to 24 h S. pneumoniae infection. LOD = limit of detection. Data are pooled from three independent experiments, with cells plated in triplicate for in vitro assays. Data are displayed as mean ± SEM. For a * p = 0.0107, *** p < 0.0001, one-way ANOVA with Dunnett’s post hoc test, b from left to right *** p < 0.0001, *** p < 0.0001, p = 0.8011, one-way ANOVA with Dunnett’s post hoc test, c from left to right *** p < 0.0001, p > 0.9999, *** p < 0.0001, *** p < 0.0001, two-way ANOVA with Sidak’s post hoc test, d *** p < 0.0001, one-way ANOVA with Tukey’s post hoc test ( e ) from left to right *** p = 0.0004, p = 0.1526, Kruskal–Wallis with Dunn’s post hoc test, f from left to right p = 0.9344, p = 0.1490, p > 0.9999, p > 0.9999, Kruskal–Wallis with Dunn’s post hoc test. Source data are provided as a Source Data file. Full size image Lipoproteins, a component of the cell membrane in both Gram-negative and Gram-positive bacteria, are the primary bacterial TLR2 ligand [37] . In contrast, TLR4 is responsive to LPS [38] . We purified lipoproteins and LPS from P. melaninogenica and found that P. melaninogenica lipoproteins, but not P. melaninogenica LPS, induced neutrophil TNFα secretion in a TLR2-dependent manner (Fig. 5c ). The digestion of bacterial lipoproteins with lipoprotein lipase abrogates TLR2 activation [39] . We found that lipoprotein lipase digestion of P. melaninogenica resulted in significant loss of neutrophil TNFα secretion in vitro (Fig. 5d ). Lipoprotein lipase-treated P. melaninogenica was also no longer protective against S. pneumoniae infection in mice (Fig. 5e ). However, lipoprotein-TLR2 signaling was not sufficient for protection, as neither the TLR2 agonist Pam3SK4 nor purified P. melaninogenica lipoproteins altered lung burdens of S. pneumoniae compared to mice treated with PBS (Fig. 5f ). Together, these findings indicate that P. melaninogenica lipoproteins activate TLR2-dependent secretion of TNFα in neutrophils and are required, but not sufficient, for P. melaninogenica -mediated protection against S. pneumoniae . TLR2 is required for P. melaninogenica -mediated protection We next addressed the importance of TLR2 for P. melaninogenica- induced immune activation and protection in vivo. In Tlr2 −/− mice exposed to P. melaninogenica HK alone (uninfected), the recruitment of both neutrophils and inflammatory monocytes was similar to that in WT mice (Fig. 6a and Supplementary Fig. 5a, b ), and CD11b hi DC and AM populations were unaffected (Supplementary Fig. 5c, d ). However, P. melaninogenica- induced neutrophil TNFα was lost in Tlr2 −/− mice (Fig. 6b ). These findings indicate that TLR2 is required for P. melaninogenica- induced neutrophil TNFα, but not P. melaninogenica- induced myeloid cell recruitment. Fig. 6: TLR2 is required for P. melaninogenica ( P. mel . )-induced neutrophil TNFα and protection against S. pneumoniae . a , b Percentage of neutrophils ( a ), representative flow cytometry plots and total cell numbers of neutrophil TNFα ( b ) detected by intracellular flow cytometry in WT or Tlr2 -/- mice treated with either PBS (-) or P. mel . strain 25845 heat-killed (HK) i.t. for 24 h ( n = 5 mice/group). c – f Lung type 2 S. pneumoniae burdens ( n = 9 mice/group) ( c ), percentage of neutrophils ( n = 5 mice/group) ( d ), percentage of inflammatory monocytes ( n = 5 mice/group) ( e ), and percentage of neutrophil TNFα ( n = 5 mice/group) ( f ) detected by intracellular flow cytometry in mice treated with either PBS (-) or P. melaninogenica ( P. mel .) HK i.t. prior to 24 h S. pneumoniae infection, 5 × 10 6 CFU/mouse. LOD = limit of detection. Data are pooled from three independent experiments ( c ) or representative from one of four independent experiments ( a , b , d – f ), displayed as mean ± SEM. For a ** p = 0.0026 (WT), ** p = 0.009 ( Tlr2 -/- ), one-way ANOVA with Sidak’s post hoc test and p = 0.0338 (WT), p = .0081 ( Tlr2 -/- ), Kruskal–Wallis with Dunn’s post hoc test, b *** p = 0.0002 (WT), p = 0.9858 ( Tlr2 -/- ), one-way ANOVA with Sidak’s post hoc test and p = 0.0165 (WT), p > 0.9999 ( Tlr2 -/- ), Kruskal–Wallis with Dunn’s post hoc test, c from left to right ** p = 0.0017, p > 0.9999, p > 0.9999, Kruskal–Wallis with Dunn’s post hoc test, d * p = 0.0494 (WT), p > 0.9999 ( Tlr2 -/- ), Kruskal–Wallis with Dunn’s post hoc test, e ** p = 0.0014 (WT), ** p = 0.0026 ( Tlr2 -/- ), one-way ANOVA with Sidak’s post hoc test and p = 0.0162 (WT), p = 0.0400 ( Tlr2 -/- ), Kruskal–Wallis with Dunn’s post hoc test, f * p = 0.0142 (WT), p = 0.9898 ( Tlr2 -/- ), one-way ANOVA with Sidak’s post hoc test and p = 0.2056 (WT), p > 0.9999 ( Tlr2 -/- ), Kruskal–Wallis with Dunn’s post hoc test. Source data are provided as a Source Data file. Full size image In Tlr2 −/− mice infected with S. pneumoniae , lung burdens were elevated regardless of Prevotella exposure, in contrast to WT mice in which Prevotella exposure was protective (Fig. 6c ). P. melaninogenica -induced neutrophil recruitment was lost in Tlr2 −/− mice infected with S. pneumoniae , while the recruitment of inflammatory monocytes was maintained (Fig. 6d, e and Supplementary Fig. 5e, f ). These data indicate that Prevotella -induced neutrophil recruitment is TLR2-dependent in S. pneumoniae -infected mice, a setting which may require TNFα feedback. Neutrophils in the lungs of Tlr2 −/− infected mice also no longer expressed TNFα in response to P. melaninogenica (Fig. 6f ). The proportions of other lung myeloid cells, including CD11b hi DCs and AMs, were similar between WT and Tlr2 −/− mice infected with S. pneumoniae (Supplementary Fig. 5g, h ). Together, these data indicate a critical role for TLR2 in P. melaninogenica- induced neutrophil activation and protection against S. pneumoniae . The separation between neutrophil expression of TNFα, which was TLR2-dependent, and the recruitment of neutrophils and inflammatory monocytes, which were TLR2-independent in P. melaninogenica -exposed mice, indicate that myeloid cell recruitment is by itself insufficient to improve protection against S. pneumoniae , which requires the activation of cells including neutrophils. P. melaninogenica enhances serine protease-mediated killing To address whether neutrophils activated by P. melaninogenica directly contribute to enhanced clearance of S. pneumoniae , neutrophil killing of S. pneumoniae was measured in vitro. Neutrophils purified from the bone marrow of naïve mice were no better at killing S. pneumoniae following pre-incubation with P. melaninogenica HK for up to 6 h (Supplementary Fig. 6a ), after which the viability of primary neutrophils declines. This suggests that while direct exposure to P. melaninogenica induces neutrophil secretion of TNFα, it is not sufficient to enhance killing of S. pneumoniae within this timeframe. We next considered whether additional cells or signals in the lungs of P. melaninogenica- exposed mice promote neutrophil killing of S. pneumoniae . To address this, neutrophils were purified from the lungs of mice exposed to either P. melaninogenica or E. coli LPS for 24 h (Fig. 7a ). E. coli LPS was chosen as a non-protective immune stimulus that would still induce neutrophil recruitment. Neutrophils purified from the lungs of Prevotella -exposed mice killed significantly more S. pneumoniae than neutrophils purified from the lungs of mice exposed to E. coli LPS (Fig. 7b ). 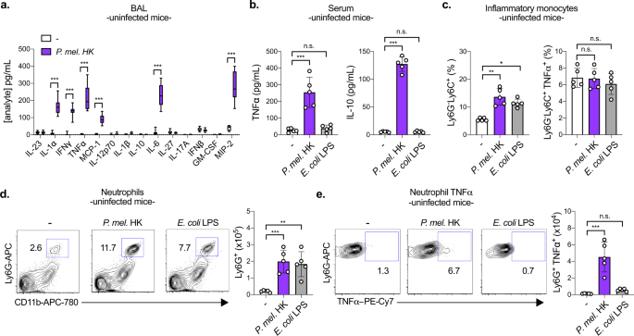Fig. 2:P. melaninogenica(P. mel.)induces a pro-inflammatory immune response in the lung associated with neutrophil activation in the absence ofS. pneumoniaeinfection. aQuantification of cytokines and chemokines in lung bronchoalveolar lavage (BAL) following exposure to PBS (-) orP. mel. heat-killed (HK) strain 25845 i.t. for 24 h (n= 10 mice/group).bSerum cytokines detected in mice exposed to PBS (-),P. mel. HK, orE. colilipopolysaccharide (LPS) i.t. for 24 h (n= 5 mice/group).c–ePercentage and total number of inflammatory monocytes (CD45+SiglecF-Ly6G-Ly6C+CD11b+cells) (c), neutrophils (CD45+SiglecF-Ly6G+CD11b+cells) (d), and neutrophil TNFα (e) detected in the lungs of mice frombby intracellular flow cytometry, with representative plots shown for the percentage of neutrophils and neutrophil TNFα (n= 5 mice/group). Data are pooled from three independent experiments (a) or representative from one of four independent experiments (b–e). Box boundaries inaindicate the 25th and 75th percentiles, with a horizontal line representing the median and whiskers indicating minimum and maximum values. Data inb–eare displayed as mean ± SEM. Fora***p< 0.0001, two-way ANOVA with Sidak’s post hoc test,bfrom left to right ***p< 0.0001,p= 0.9108 (TNFα), ***p< 0.0001,p= 0.9108 (IL-10), one-way ANOVA with Dunnett’s post hoc test and from left to rightp= 0.0060,p> 0.9999 (TNFα),p= 0.0144,p> 0.9999 (IL-10), Kruskal–Wallis with Dunn’s post hoc test,cfrom left to right **p= 0.0044, *p= 0.0453,p= 0.9875,p= 0.5395, Kruskal–Wallis with Dunn’s post hoc test,dfrom left to right ***p= 0.009, **p= 0.0017, one-way ANOVA with Dunnett’s post hoc test andp= 0.0115,p= 0.0215, Kruskal–Wallis with Dunn’s post hoc test,efrom left to right ***p< 0.0001,p= 0.7296, one-way ANOVA with Dunnett’s post hoc test andp= 0.0008,p= 0.1542, Kruskal–Wallis with Dunn’s post hoc test. Source data areprovided as a Source Data file. The two primary mechanisms for neutrophil killing of S. pneumoniae are the production of reactive oxygen species (ROS) and activity of serine proteases. Neutrophils from P. melaninogenica- exposed and E. coli LPS-exposed mice produced similar levels of total ROS (Fig. 7c ). In contrast, the activity of two serine proteases, cathepsin G and elastase, was significantly higher in neutrophils purified from the lungs of P. melaninogenica -exposed mice, compared to neutrophils from the lungs of mice exposed to E. coli LPS (Fig. 7d ). Neutrophils pooled from naïve mice had similarly low serine protease activity as those from E. coli LPS-exposed mice (Supplementary Fig. 6b ). The addition of protease inhibitors, but not the ROS inhibitor DPI, significantly reduced S. pneumoniae killing by neutrophils isolated from P. melaninogenica -exposed mice (Fig. 7e ), without affecting S. pneumoniae growth (Supplementary Fig. 6c ). These data indicate that serine protease activity is important for P. melaninogenica -enhanced killing in lung neutrophils. Fig. 7: P. melaninogenica ( P. mel .) enhances serine protease-mediated killing of S. pneumoniae by lung neutrophils in a TLR2-dependent manner. a Schematic of lung neutrophil purification. b Percent of type 2 S. pneumoniae killed by lung neutrophils purified from mice exposed to either E. coli lipopolysaccharide (LPS) or P. mel . strain 25845 heat-killed (HK) i.t. for 24 h following 1 h incubation with S. pneumoniae opsonized with 3% fresh mouse serum ( n = cells isolated from 11 mice/group). c Total reactive oxygen species (ROS) produced in 1 h by lung neutrophils purified from mice exposed to either E. coli LPS or P. mel . HK i.t. for 24 h detected by luminol, with area under curve (AUC) shown ( n = cells isolated from 6 mice/group). d Serine protease activity for cathepsin G and elastase + /– protease inhibitor cocktail (Prot Inhib) detected by substrate cleavage for lung neutrophils purified from WT mice exposed to either E. coli LPS or P. mel . HK ( n = cells isolated from 6 mice/group). e Percent of S. pneumoniae killed by lung neutrophils purified from WT mice exposed to P. mel . HK i.t. for 24 h following 1 h incubation with opsonized S. pneumoniae in the presence of the ROS inhibitor DPI (ROS), protease inhibitors (Protease), or no inhibitors (none), ( n = cells isolated from 9 mice/group). f , g Percent of S. pneumoniae killed by lung neutrophils purified from WT or Tlr2 -/- mice exposed to P. mel . HK i.t. for 24 h ( n = cells isolated from 13 WT mice, 9 Tlr2 -/- mice) ( f ) or serine protease activity +/– protease inhibitor cocktail (Prot Inhib) ( n = cells isolated from 6 mice/group) ( g ). Data are pooled from three independent experiments, with cells plated in duplicate or triplicate. Data are displayed as mean ± SEM. For b *** p < 0.0001, two-tailed t -test, c p = 0.9566, two-tailed t -test, d *** p = 0.0004 (Cathepsin G), *** p < 0.0001 (Elastase), two-tailed t -test, e p = 0.9926 (ROS), *** p < 0.0001 (Protease), one-way ANOVA with Dunnett’s post hoc test, f *** p < 0.0001, two-tailed t -test, g *** p = 0.0008 (Cathepsin G), *** p = 0.0002 (Elastase), two-tailed t -test. Source data are provided as a Source Data file. Full size image The importance of TLR2 signaling for Prevotella -induced neutrophil killing was determined by comparing neutrophils purified from WT versus Tlr2 −/− mice. Neutrophils from the lungs of Tlr2 −/− mice exposed to P. melaninogenica were less efficient at killing S. pneumoniae compared to those from WT mice (Fig. 7f ) and these cells had negligible serine protease activity (Fig. 7g ), demonstrating a critical role for TLR2 in P. melaninogenica- enhanced neutrophil killing. Together, these findings suggest that P. melaninogenica exposure increases TLR2-dependent, serine protease-mediated killing of S. pneumoniae by lung neutrophils. P. melaninogenica protection requires regulation by IL-10 Immune regulation is critical to mitigate the damaging effects of inflammation in the lung such as barrier disruption and reduced oxygen exchange. While TNFα primes several protective immune responses, overproduction causes tissue damage and impairs S. pneumoniae clearance [40] , [41] . The anti-inflammatory cytokine IL-10 is a master regulator of pro-inflammatory responses including TNFα [42] . In purified neutrophils, we found that in addition to TNFα, P. melaninogenica HK induced the secretion of IL-10 in a dose-dependent and TLR2-dependent manner (Supplementary Fig. 7a ). Further, neutrophil secretion of TNFα was inhibited in cultures exposed to both P. melaninogenica and S. pneumoniae , suggesting regulation of this response (Supplementary Fig. 7b ). These findings mirror the systemic TNFα response in Prevotella -exposed mice, which was reduced following S. pneumoniae infection. Additionally, P. melaninogenica- exposed mice infected with S. pneumoniae had significantly reduced levels of several pro-inflammatory cytokines in lung BAL, including TNFα, IL-6, IL-1α, IFNβ, and IFNγ, compared to those infected with S. pneumoniae but not exposed to Prevotella (Fig. 8a ). This is in contrast to uninfected mice, where P. melaninogenica exposure increased BAL pro-inflammatory cytokines at 24 h, indicating that by 48 h in co-infected mice, these responses were reduced. These data suggest that exposure to P. melaninogenica regulates S. pneumoniae -induced inflammation in the lung. Fig. 8: P. melaninogenica ( P. mel .) - mediated protection against S. pneumoniae requires restraint of detrimental inflammation by IL-10. a Quantification of cytokines and chemokines in lung bronchoalveolar lavage (BAL) following exposure to PBS (-) or P. mel . strain 25845 heat-killed (HK) i.t. prior to 24 h type 2 S. pneumoniae infection, 5 × 10 6 CFU/mouse ( n = 9 mice/group). b , c Lung S. pneumoniae burdens ( b ) and serum TNFα ( c ) detected in WT or Il10 -/- mice exposed to either PBS (-) or P. mel . HK i.t. prior to 24 h S. pneumoniae infection ( n = 5 mice/group). d – f Representative flow cytometry plots and total cell numbers of neutrophil TNFα ( d ), percentage of inflammatory monocyte TNFα ( e ), and percentage of AM TNFα ( f ) detected by intracellular flow cytometry from WT or Il10 -/- mice treated with either PBS (-) or P. mel . HK i.t. prior to 24 h S. pneumoniae infection ( n = 4 mice/group). LOD = limit of detection. Data are pooled from three independent experiments ( a ) or representative from one of four independent experiments ( b – f ). Box boundaries in ( a ) indicate the 25th and 75th percentiles, with a horizontal line representing the median and whiskers indicating minimum and maximum values. Data in b – f are displayed as mean ± SEM. For a *** p < 0.0001, two-way ANOVA with Sidak’s post hoc test, b * p = 0.0257 (WT), p > 0.9999 ( Il10 -/- ), Kruskal–Wallis with Dunn’s post hoc test, c from left to right * p = 0.0393, p = 0.9973, ** p = 0.0012, one-way ANOVA with Tukey’s post hoc test, d from left to right * p = 0.0116, p = 0.7388, one-way ANOVA with Sidak’s post hoc test ( e ), from left to right * p = 0.0101, p = 0.1698, one-way ANOVA with Sidak’s post hoc test, f from left to right * p = 0.0280, p = 0.9298, one-way ANOVA with Sidak’s post hoc test. Source data are provided as a Source Data file. Full size image To address the potential role of regulatory IL-10 in P. melaninogenica -exposed mice, we compared S. pneumoniae burdens in WT and IL-10 deficient ( Il10 −/− ) mice with and without pre-exposure to P. melaninogenica HK. Unexpectedly, P. melaninogenica -mediated protection against S. pneumoniae was lost in Il10 −/− mice, which had similarly high burdens regardless of P. melaninogenica exposure (Fig. 8b ). In Il10 −/− mice, serum TNFα was elevated following P. melaninogenica exposure (Fig. 8c ). In contrast, WT mice exposed to P. melaninogenica had reduced serum TNFα and elevated IL-10 (Supplementary Fig. 7c ). These results indicate that P. melaninogenica -induced IL-10 regulates systemic TNFα during S. pneumoniae infection and is important for P. melaninogenica- mediated protection. Analysis of lung myeloid cell TNFα expression revealed that TNFα was significantly elevated in several cell types, including neutrophils, inflammatory monocytes, and AMs, in Il10 −/− mice, regardless of P. melaninogenica exposure (Fig. 8d–f and Supplementary Fig. 7d–e ). Depletion of TNFα was not sufficient to reverse the loss of P. melaninogenica -mediated protection in Il10 −/− mice (Supplementary Fig. 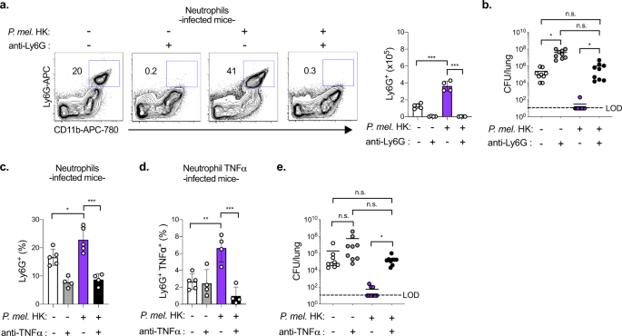Fig. 3: Neutrophils and TNFα are critical forP. melaninogenica(P. mel.)-mediated protection againstS. pneumoniaeinfection. a,bRepresentative flow cytometry plots and total cell numbers for neutrophils detected by flow cytometry (n= 5 mice/group, PBS, n = 4 mice/group, others) (a) and lung burdens of type 2S. pneumoniae(n= 9 mice/group) (b) in mice treated with isotype control or anti-Ly6G antibodies (200 μg/mouse) i.p. together with either PBS (-) orP. mel. strain 25845 heat-killed (HK) i.t. prior to 24 hS. pneumoniaeinfection, 5×106CFU/mouse.c–eTotal cell number of neutrophils and neutrophil TNFα detected by intracellular flow cytometry (n= 5 mice/group for isotype control groups, 4 mice/group for anti-TNFα groups) (c,d) and lungS. pneumoniaeburdens (n= 9 mice/group) (e) in mice treated with isotype control or anti-TNFα antibodies (200 μg/mouse) i.p. together with either PBS (-) orP. mel. HK i.t. prior to 24 hS. pneumoniaeinfection. LOD = limit of detection. Data are pooled from three independent experiments (b,e) or representative from one of four independent experiments (a,c,d), displayed as mean ± SEM. Fora***p< 0.0001, one-way ANOVA with Sidak’s post hoc test,bfrom left to right *p= 0.0222,p> 0.9999,p= 0.0751, *p= 0.0192, Kruskal–Wallis with Dunn’s post hoc test,cfrom left to right *p= 0.0337, ***p< 0.0001 one-way ANOVA with Tukey’s post hoc test,d**p= 0.003, ***p= 0.0002 one-way ANOVA with Tukey’s post hoc test,efrom left to rightp= 0.3058,p> 0.9999,p= 0.4470, *p= 0.0118, Kruskal–Wallis with Dunn’s post hoc test. Source data are provided as a Source Data file. 7f ), suggesting a broad loss of IL-10-mediated restraint of myeloid cell activation. Together, these findings reveal that IL-10 regulation of lung inflammation is a critical component of P. melaninogenica -mediated protection against S. pneumoniae infection. Protection mediated by other airway Prevotella While P. melaninogenica is an abundant Prevotella species, it was unclear whether other airway Prevotella isolates mediate a similar protective effect. As with P. melaninogenica strain 25845, used throughout these studies, exposure to live P. melaninogenica strain D18 significantly improved clearance of S. pneumoniae from the lung by 24 h post-infection (Fig. 9a ). Three additional live airway Prevotella species, including Prevotella buccae , Prevotella tannerae , and Prevotella nanceiensis , also increased S. pneumoniae clearance from the lung (Fig. 9a ). In contrast, the periodontal pathogen P. intermedia was not protective (Fig. 9a ). These data suggest that several airway Prevotella species are capable of enhancing protection against S. pneumoniae infection. Finally, we compared the ability of HK preparations of each Prevotella species to activate neutrophils purified from the bone marrow of WT versus Tlr2 −/− mice. Similar to P. melaninogenica strain 25845, strain D18 as well as P. buccae , P. tannerae , and P. nanceiensis induced neutrophil secretion of TNFα and IL-10 in a TLR2-dependent manner (Fig. 9b ). In contrast, P. intermedia activated neutrophils in a TLR2-independent manner (Fig. 9b ). These data are consistent with a critical role for TLR2-dependent neutrophil activation in species of Prevotella which are protective against S. pneumoniae . Fig. 9: Protection against S. pneumoniae is induced by other airway Prevotella that activate neutrophils in a TLR2-dependent manner. a Lung S. pneumoniae burdens in mice treated with PBS (-), live P. melaninogenica ( P. mel .) strain D18, live P. buccae , live P. tannerae , live P. nanceiensis , or live P. intermedia i.t. prior to 24 h S. pneumoniae infection, 5 × 10 6 CFU/mouse ( n = 12 mice/group). b Supernatant cytokines detected 24 h following incubation of BM neutrophils with P. mel . strain D18 heat-killed (HK), P. buccae HK, P. tannerae HK, P. nanceiensis HK, or P. intermedia HK ( n = 3 independent experiments/group). Data are pooled from three independent experiments, with cells plated in triplicate for in vitro studies, displayed as mean ± SEM. For a from left to right *** p < 0.0001, *** p < 0.0001, *** p = 0.0005, *** p < 0.0001, p = 0.9999, Kruskal–Wallis with Dunn’s post hoc test, b from left to right, *** p < 0.0001, *** p < 0.0001, *** p < 0.0001, *** p < 0.0001, p = 0.9959 (TNFα), *** p < 0.0001, *** p < 0.0001, *** p < 0.0001, *** p < 0.0001, p = 0.9948 (IL-10), two-way ANOVA with Sidak’s post hoc test. Source data are provided as a Source Data file. Full size image Work over the past decade has defined the gut-lung axis, highlighting a critical role for the gut microbiome in lung immune homeostasis. By comparison, our understanding of immune regulation by members of the airway microbiome is underdeveloped. Several individual members of the respiratory tract microbiome, including commensal Streptococcus and Corynebacterium species, produce factors that inhibit growth of S. pneumoniae [28] , [29] , [30] . However, it is less clear how these and other airway commensals regulate innate immune-mediated protection against lung infection [43] . Brown et al. showed that a compilation of Gram-positive airway bacteria including Lactobacillus crispatus, Staphylococcus aureus , and Staphylococcus epidermidis induced Nod2-dependent protection against S. pneumoniae [8] . In this case, a Nod2-activating bacterial cohort from the gut also induced protection, which required GM-CSF and AMs. As we did not detect a GM-CSF response to Prevotella , this suggests there are at least two distinct microbial-induced immune pathways capable of enhancing protection against S. pneumoniae . Sustained protection against S. pneumoniae infection in antibiotic treated and Germ-free mice indicates that P. melaninogenica is sufficient to drive immune-mediated protection without the participation of other members of the endogenous microbiota. This study focused on the early response to P. melaninogenica in the context of acute lung infection. Recently, a compilation of oral commensals which included P. melaninogenica was shown to protect against S. pneumoniae for as long as 2 weeks [44] . Protection at this timepoint was associated with the induction of a Th17 response, which correlated primarily with the presence of Veillonella rather than Prevotella . However, RNA sequencing of lung tissue 24 h post-commensal aspiration confirmed the induction of TLR signaling and inflammatory responses including TNFα and IL-6, similar to our findings with P. melaninogenica . This indicates that exposure to either P. melaninogenica alone or in combination with other oral commensals enhances immune-mediated protection against S. pneumoniae . Prevotella -induced immune responses may coordinate with those induced by other commensal bacteria, such as Veillonella , for extended protection. Inflammation itself is not automatically protective against S. pneumoniae infection. For example, virus-induced inflammation supports increased S. pneumoniae growth [45] , and viral-pneumococcal co-infections are associated with higher morbidity and mortality [46] . Similarly, S. pneumoniae co-infection with H. influenzae involves synergistic inflammation, including the upregulation of TLR2 signaling in the lung and middle ear. S. pneumoniae is well-equipped for immune modulation and evasion, and expresses virulence factors that limit the efficacy of innate immune responses and impede neutrophil-mediated killing [47] , [48] . As a result, innate immune cells are typically insufficient for pneumococcal clearance. Our findings highlight a protective role for TLR2-dependent inflammation induced by airway Prevotella exposure, the timing of which may be important for overcoming S. pneumoniae immune evasion mechanisms. This may relate to reduced acquisition of S. pneumoniae in the lungs of individuals with “optimal” innate immune priming by their airway microbiota. The concept of trained immunity refers to non-specific beneficial immune priming, primarily mediated by innate immune signaling and directed by the microbiota. The critical cells and signaling pathways in the lung for trained immunity are not clear. Compared with all other tissues including the gut, the lungs have the highest expression of TLR2 [49] . Immune priming by TLR agonists has been explored as a potential immunotherapy strategy for several infections, including S. pneumoniae . Specific combinations of TLR agonists are protective against S. pneumoniae infection, such as TLR2 together with TLR9 agonists [50] . S. pneumoniae lipoproteins are capable of activating TLR2 [51] , similar to Prevotella , but TLR2 is not sufficient for protection [52] , as we confirm. One study, however, found that TLR2 is protective against pneumolysin-deficient S. pneumoniae , which no longer activates TLR4 [53] . Prevotella express penta-acylated LPS, which can behave as a TLR4 agonist, in contrast to hexa-acylated LPS expressed by bacteria such as E. coli , which is a strong TLR4-inducer [54] . Further investigation is required to dissect the immune priming environment which coordinates with TLR2 to promote P. melaninogenica -mediated protection against S. pneumoniae , including the potential role of TLR4 antagonism. The protective capacity of TLR priming also differs by infection, as TLR4 priming with E. coli -derived LPS improves protection against lung infection with Klebsiella pneumoniae and influenza A virus [31] , [32] , in contrast to S. pneumoniae . Together, these studies highlight the importance of understanding the context and mechanism of protective airway microbiome trained immunity. While our data indicate an important role for neutrophils, it remains unclear which cells initiate neutrophil recruitment in response to P. melaninogenica . AMs are a likely candidate as the first immune cells to encounter inhaled particles and as a major source of neutrophil chemoattractants [33] . P. melaninogenica outer membrane vesicles induce AM responses including IL-17A and IL-17B [27] , which can synergize with pro-inflammatory cytokines including TNFα. As others have shown [55] , we find that TNFα is important for neutrophil recruitment during S. pneumoniae infection, and TNFα can prime activation of human neutrophils [56] . However, TNFα priming in neutrophils is typically associated with stronger NADPH oxidase activation and respiratory burst [57] . This contrasts with our findings of increased serine protease activity, which was dependent on additional signals in the P. melaninogenica -activated lung. Serine protease activity is essential for neutrophil killing of S. pneumoniae [58] , and serine protease knockout mice have reduced clearance of S. pneumoniae from the lung [59] , highlighting the importance of this pathway for infection control. Here, we find that Prevotella -mediated protection requires the co-induction of systemic IL-10, which regulates Prevotella -induced inflammation in S. pneumoniae -infected mice. In contrast to this beneficial role, we recently found that systemic IL-10 induced at 3 days post-infection exacerbates S. pneumoniae lung infection [60] . However, this response was delayed relative to the protective IL-10 response we observe in Prevotella -exposed mice. Others have shown that P. melaninogenica induces the production of IL-10 by human DCs [61] , and we find that murine neutrophils secrete IL-10 in response to P. melaninogenica , suggesting that myeloid cell-derived IL-10 contributes to inflammatory control. These studies highlight the importance of inflammatory fine-tuning in the lung, where IL-10 plays a major role in limiting tissue damage, though at the risk of worsened infection under some circumstances. Despite the genetic heterogeneity reported among Prevotella species [62] , we identified two different isolates of P. melaninogenica and several other airway Prevotella species that enhance protection against S. pneumoniae . P. melaninogenica was previously shown to induce similar immune activation profiles, including the production of TNFα and IL-10 by lung CD45 + cells, as P. nanceiensis [22] , one of the strains we identify as protective. Although not as prevalent as P. melaninogenica , P. buccae , P. tannerae , and P. nanceiensis are also common in the upper and lower airway of healthy individuals [4] , [63] . In contrast, P. intermedia , which was not protective against S. pneumoniae , is a major periodontal pathogen. Others have reported that P. intermedia upregulates a critical adherence receptor used by S. pneumoniae in airway epithelial cells, exacerbating type 4 S. pneumoniae infection [25] . Here, we find that P. intermedia activates neutrophils in a TLR2-independent manner, unlike the other Prevotella strains, which are protective. The critical features of protective airway Prevotella species, including the role of TLR2-dependent neutrophil activation and regulation of the airway epithelium, is an important area for further investigation. Regardless, these findings suggest that the species-specific composition of airway Prevotella dictates infection outcome following S. pneumoniae exposure. The immune activation profile we describe is consistent with several observations in humans, including the association between increased Prevotella and sub-clinical inflammation characterized by increased neutrophils, the human neutrophil chemotactic factor IL-8, Mip-1α, and IL-10 in the lungs of healthy adults [20] , [64] . Similarly, Prevotella abundance was associated with increased TNFα and IL-10 in the lungs of transplant patients, in whom Prevotella correlated with increased lung function and airway microbiome stability [19] . Finally, in vitro studies demonstrate the capacity of P. melaninogenica to induce TLR2 activation and responses including IL-6, TNFα, and IL-10 secretion by human monocytes and DCs [61] , [65] , [66] . Together, these findings indicate that Prevotella species including P. melaninogenica are associated with lung innate immune responses including TLR2 activation and the production of TNFα and IL-10 in both humans and animal models. Our findings highlight an important role for airway Prevotella in directing immune-mediated protection in the respiratory tract. Further studies will be necessary to determine whether similar protective immune priming is induced by Prevotella aspiration in healthy adults and how such protection may be leveraged to reduce the burden of lung infections in susceptible individuals. Airway immunobiotics, or probiotics designed to enhance protective immunity, may be particularly impactful in individuals who are at increased risk of S. pneumoniae infection, though such use should be tempered by potentially detrimental effects, for example by exacerbating fibrosis in those with chronic lung disease. Alternatively, targeting the critical Prevotella -modified immune pathways could improve clearance of S. pneumoniae regardless of the presence of Prevotella as an immunotherapeutic strategy. Animals Adult male and female mice aged 6-12 weeks of age were used for these studies. C57BL/6 J (WT), B6.129Tlr2 tm1Kir ( Tlr2 −/− ), and B6.129il10 tm1Cgn ( Il10 −/− ) mice were purchased from The Jackson Laboratory (stocks #000664, 004650, and 002251 respectively). All strains used in these studies (WT, Tlr2 −/− and Il10 −/− ) are on the C57BL/6J genetic background. Mice were maintained in the University of Colorado Office of Laboratory Animal Resources. Housing conditions included a light cycle of 14:10 (light:dark) hours, a temperature of 72 ± 2°F, with 40 ± 10% humidity. Mice were fed irradiated Tecklad diet (Envigo, Inotiv, Inc.), catalog #2920X for colony mice and #2919 for breeder pairs. Germ-free mice were obtained from the University of Colorado Anschutz Medical Campus Gnotobiotic Facility, which maintains a colony established with founder C57BL/6 mice obtained from the National Gnotobiotic Rodent Resource Center at the University of North Carolina. Germ-free mice are housed in sterilized vinyl film isolators with positive pressure air flow through HEPA filtration. Any items introduced into the isolators are sterilized, with quality control indicators to verify sterilization. The internal isolator environment and housed mice are tested bi-weekly and prior to experimental use for microbiota through culture-dependent methods and by qPCR (see Microbiome Depletion). For infection experiments, Germ-free mice were transferred directly from the Gnotobiotic Core Facility into BSL2 vivarium space. Transferred mice were exposed to input bacteria (see Infections) within 8 h of transfer. Microbiome depletion Antibiotic treated mice were exposed to a broad-spectrum antibiotic cocktail (ampicillin 1 g/L, neomycin 1 g/L, metronidazole 1 g/L, vancomycin 0.5 g/L, MilliporeSigma and McKesson) in drinking water ad libitum for 7 days. Water containing antibiotics was replaced with normal drinking water 48 h prior to live Prevotella exposure. Microbiome depletion was confirmed by qPCR using genomic DNA extracted from stool samples using the PureLink™ Genomic DNA Mini Kit (ThermoFisher Scientific). Primers (ACTCCTACGGGAGGCAGCAGT and ATTACCGCGGCTGCTGGC) were used with iTaq™ Universal SYBR ® Green Supermix (BioRad) and 1 μL template DNA, with reactions performed on a CFX Connect™ Real-Time System (BioRad) under the following cycle conditions: (1) 94 °C 4 min; (2) 40 cycles of 15 s at 95 °C, 30 s at 60 °C, and (3) 72 °C for 10 min. Total 16 S rRNA gene copy numbers were calculated using a standard curve generated with a known concentration of S. pneumoniae D39 gDNA, input ng/μL DNA, and Ct values. qPCR data were analyzed using CFX Manager Software (version 2.1, BioRad). Bacteria Prevotella melaninogenica strain ATCC ® 25845™, Prevotella tannerae strain ATCC ® 51259™, and Prevotella intermedia strain ATCC ® 25611™ were obtained from the American Type Culture Collection, Manassas VA. Prevotella melaninogenica strain D18 (catalog #HM-80) and Prevotella buccae strain D17 (catalog #HM-45) were obtained from BEI resources, NIAID, NIH as part of the Human Microbiome project. Prevotella nanceiensis strain PP1746 was a kind gift from Dr. Paul Planet, Division of Infectious Diseases at the Children’s Hospital of Philadelphia. Prevotella strains were grown under anaerobic conditions on Brucella Agar containing 5% sheep blood, hemin and vitamin K at 37 °C for 72 h (ThermoFisher Scientific). Heat-killed Prevotella were prepared from fresh plates following resuspension in PBS and incubation at 56 °C for 35 min. Samples before and after heat-killing were used to determine CFU equivalents/mL and confirm killing, respectively. Heat-killed Corynebacterium accolens strain ATCC ® 49726™ (American Type Culture Collection) and Corynebacterium amycolatum strain SK46, catalog #HM-109 (BEI resources, NIAID, NIH as part of the Human Microbiome project) were prepared following growth in BHI broth cultures supplemented with 1% Tween ® 80 (polysorbate, VWR). Heat-killed Streptococcus salivarius strain SK126, catalog #HM-109 (obtained from BEI Resources, NIAID, NIH as part of the Human Microbiome project) was prepared following growth in Todd Hewitt Broth with 5% Yeast Extract (BD Bacto™) at 37 °C with 5% CO 2 without shaking. Heat-killed Escherichia coli (strain DH5α, ThermoFisher Scientific) was prepared following growth in LB broth (BD Bacto™) at 37 °C with shaking (200 rpm). A streptomycin resistant variant of serotype 2 Streptococcus pneumoniae strain D39 was a kind gift from Dr. Jeffrey N. Weiser (New York University). Serotype 3 S. pneumoniae strain ATCC ® 6303™ (American Type Culture Collection) was also used. S. pneumoniae was grown in Todd Hewitt Broth with 5% Yeast Extract (BD Bacto™), with 50 μg/mL streptomycin (Sigma), added for type 2 strain D39 only, at 37 °C with 5% CO 2 without shaking. Infections For live P. melaninogenica infections, bacterial suspensions from fresh plates were prepared in PBS to an optical density (OD 600 ) of 0.3, centrifuged at ≥20,000 x g for 10 min, and resuspended in PBS prior to injection. S. pneumoniae was grown in broth from frozen stocks to mid-log phase and centrifuged at ≥20,000 x g for 10 min followed by resuspension in PBS for infections. Inoculum burdens were determined by serial dilution for CFU enumeration. Lungs and spleens collected from infected mice were homogenized using a Bullet Blender tissue homogenizer (Stellar Scientific, Baltimore, MD). Tissue burdens were calculated following serial dilution in PBS and growth on Tryptic Soy agar plates containing neomycin (5 μg/mL, Sigma) and streptomycin (50 μg/mL, D39 STR strain only) prepared with fresh catalase (5000 Units/plate, Worthington Biochemical Corporation, Lakewood, NJ). Plates were grown at 37 °C with 5% CO 2 for 24 h. All intratracheal and intranasal infections were conducted in a volume of 50 μL on mice anesthetized by inhaled isoflurane. For cell and cytokine depletions, mice were treated intraperitoneally 24 h prior to S. pneumoniae infection with 200 μg/mouse isotype control anti-IgG2A antibody (clone C1.18, catalog #BE0085, lot #722719J2), anti-Ly6G antibody (clone 1A8, catalog #BE0071-1, lot #80772101), or anti-TNFα antibody (clone XT3.11, catalog #BE0058, lot #728221A1) as indicated (Bio X Cell, Lebanon, NH). For E. coli LPS (0111:B4, Sigma), P. melaninogenica lipoprotein (described below) and Pam3SK4 treatments, mice were treated with 10 μg (LPS) or 10–50 μg (Pam3SK4) i.t. 24 h prior to S. pneumoniae infection. For survival assays, moribund mice humanely euthanized. Flow cytometry Lungs were harvested following perfusion by transcardial injection of 10 mL PBS, and single cells were prepared for flow cytometry [60] . Briefly, lungs were subjected to mechanical (mincing) and enzymatic (DNAseI 30 μg/mL, Sigma, and type 4 collagenase 1 mg/mL, Worthington Biochemical Corporation) digestion prior to passage through a 70 μM strainer. Red blood cells were lysed in RBC lysis buffer (0.15 M NH 4 Cl, 10 mM KHC0 3 , 0.1 mM Na 2 EDTA, pH 7.4). Fc receptors were blocked by incubation in anti-CD16/32 (2.4G2 hybridoma supernatant) prior to staining in FACS buffer (1% BSA, 0.01% NaN3, PBS). For intracellular flow cytometry, cells were incubated with Brefeldin A (BD Biosciences) prior to staining and permeabilized with 1 mg/mL saponin (Sigma) prior to intracellular staining. All cells were fixed in 1% paraformaldehyde. Antibodies used for staining included anti-mouse: Siglec F (BD, catalog #562681, clone E50-2440, lot #B302914), MHCII (BioLegend, catalog #107643, clone M5/114.15.2, lot #B317262), Ly6G (BioLegend, catalog #127614, clone 1A8, lot #B292772), Ly6C (BioLegend, catalog #128012, clone HK1.4, lot #B250462), CD45.2 (BD, catalog #564616, clone 104, lot #1083734), CD11c (BioLegend, catalog #117338, clone N418, lot #B290360), CD11b (BioLegend, catalog #101212, clone M1/70, lot #B281906), and TNFα (ThermoFisher Scientific, catalog #25-7321-82, clone MP6-XT22, lot #2044683). 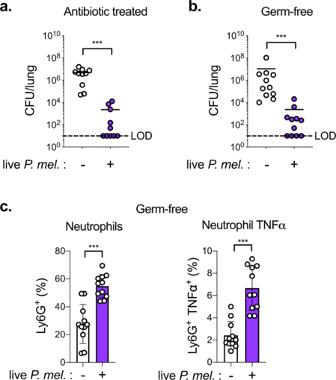Fig. 4:P. melaninogenica(P. mel.) is protective againstS. pneumoniaeinfection in microbiome-depleted mice. aLungS. pneumoniaeburdens in mice treated with antibiotics followed by exposure to PBS (-) or liveP. mel. strain 25845 i.t. prior to 24 hS. pneumoniaeinfection, 5 × 106CFU/mouse (n= 9 mice/group).b,cLungS. pneumoniaeburdens (b) and percent neutrophils, neutrophil TNFα (c) in Germ-free mice treated with either PBS (-) or liveP. mel. i.t. prior to 24 hS. pneumoniaeinfection, 106CFU/mouse (n= 11 mice/group). LOD = limit of detection. Data are pooled from three independent experiments. Data are displayed as mean ± SEM. Fora,b***p< 0.0001 two-tailed Mann–WhitneyU-test,c***p< 0.0001 two-tailedt-test. Source data are provided as a Source Data file. All antibodies were used at a 1:200 dilution for staining. Flow cytometry was performed on an LSR Fortessa X-20 in the ImmunoMicro Flow Cytometry Shared Resource Laboratory at the University of Colorado Anschutz Medical Campus (RRID:SCR_021321). Data analysis was performed using FlowJo™ Software, version 9.9.6 (BD Life Sciences). Cytokine and chemokine analysis BAL cytokines and chemokines with the exception of MIP-2 were measured using a LEGENDplex™ Mouse Inflammation Panel (BioLegend), with analytes detected on the LSR Fortessa X-20 in the ImmunoMicro Flow Cytometry Shared Resource Laboratory at the University of Colorado Anschutz Medical Campus (RRID:SCR_021321). Data were analyzed using the LEGENDplex™ Data Analysis Software Suite (BioLegend). BAL MIP-2 was measured using a mouse CXCL2/MIP-2 ELISA kit (R&D Systems), serum cytokines were measured using mouse IL-10 and TNFα ELISA kits (BD), and analytes were detected on a Synergy™ HT Microplate Reader (BioTek). 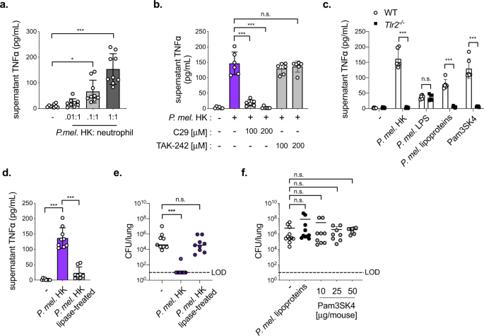Fig. 5:P. melaninogenica(P. mel.) lipoproteins induce neutrophil TNFα secretion in a TLR2-dependent manner. aSupernatant TNFα detected 24 h following incubation of bone marrow (BM) neutrophils purified from naïve wild-type (WT) mice withP. mel. strain 25845 heat-killed (HK) at the indicated ratios (n= 3 independent experiments/group).bSupernatant TNFα detected 24 h following incubation of BM neutrophils from WT mice incubated withP. mel. HK (1:1 ratio) with and without inhibitors of TLR2 (C29) or TLR4 (TAK-242), (n= 3 independent experiments/group).cSupernatant TNFα detected 24 h following incubation of BM neutrophils from WT orTlr2-/-mice with PBS (-),P. mel. HK (1:1 ratio),P. mel. lipopolysaccharide (LPS, 10 ng/mL),P. mel. lipoproteins (10 ng/mL), or Pam3SK4 (10 ng/mL), (n= 3 independent experiments/group).dSupernatant TNFα detected 24 h following incubation of BM neutrophils from WT mice treated with PBS (-), untreatedP. mel. HK, or lipoprotein-digestedP. mel. HK (n= 3 independent experiments/group).eLung type 2S. pneumoniaeburdens in mice treated with PBS (-), untreatedP. mel. HK, or lipoprotein-digestedP. mel. HK i.t. prior to 24 hS. pneumoniaeinfection, 5×106CFU/mouse (n= 9 mice/group).fLungS. pneumoniaeburdens in mice treated with PBS (-,n= 11 mice),P. mel. lipoproteins (10 μg/mouse,n= 9 mice), or Pam3SK4 (10 μg/mouse,n= 10 mice, 25 μg/mouse,n= 8 mice, or 50 μg/mouse,n= 8 mice) i.t. prior to 24 hS. pneumoniaeinfection. LOD = limit of detection. Data are pooled from three independent experiments, with cells plated in triplicate for in vitro assays. Data are displayed as mean ± SEM. Fora*p= 0.0107, ***p< 0.0001, one-way ANOVA with Dunnett’s post hoc test,bfrom left to right ***p< 0.0001, ***p< 0.0001,p= 0.8011, one-way ANOVA with Dunnett’s post hoc test,cfrom left to right ***p< 0.0001,p> 0.9999, ***p< 0.0001, ***p< 0.0001, two-way ANOVA with Sidak’s post hoc test,d***p< 0.0001, one-way ANOVA with Tukey’s post hoc test (e) from left to right ***p= 0.0004,p= 0.1526, Kruskal–Wallis with Dunn’s post hoc test,ffrom left to rightp= 0.9344,p= 0.1490,p> 0.9999,p> 0.9999, Kruskal–Wallis with Dunn’s post hoc test. Source data are provided as a Source Data file. Data were analyzed using Prism (GraphPad, version 8). 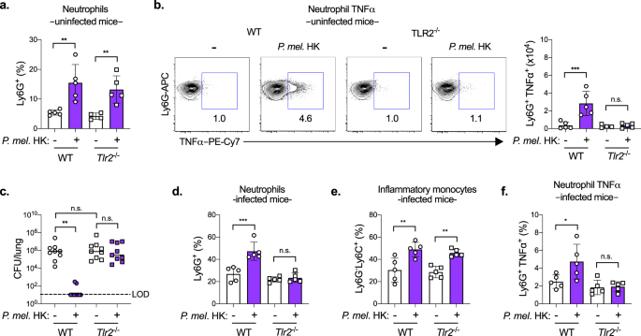Fig. 6: TLR2 is required forP. melaninogenica(P. mel.)-induced neutrophil TNFα and protection againstS. pneumoniae. a,bPercentage of neutrophils (a), representative flow cytometry plots and total cell numbers of neutrophil TNFα (b) detected by intracellular flow cytometry in WT orTlr2-/-mice treated with either PBS (-) orP. mel. strain 25845 heat-killed (HK) i.t. for 24 h (n= 5 mice/group).c–fLung type 2S. pneumoniaeburdens (n= 9 mice/group) (c), percentage of neutrophils (n= 5 mice/group) (d), percentage of inflammatory monocytes (n= 5 mice/group) (e), and percentage of neutrophil TNFα (n= 5 mice/group) (f) detected by intracellular flow cytometry in mice treated with either PBS (-) orP. melaninogenica(P. mel.) HK i.t. prior to 24 hS. pneumoniaeinfection, 5 × 106CFU/mouse. LOD = limit of detection. Data are pooled from three independent experiments (c) or representative from one of four independent experiments (a,b,d–f), displayed as mean ± SEM. Fora**p= 0.0026 (WT), **p= 0.009 (Tlr2-/-), one-way ANOVA with Sidak’s post hoc test andp= 0.0338 (WT),p= .0081 (Tlr2-/-), Kruskal–Wallis with Dunn’s post hoc test,b***p= 0.0002 (WT),p= 0.9858 (Tlr2-/-), one-way ANOVA with Sidak’s post hoc test andp= 0.0165 (WT),p> 0.9999 (Tlr2-/-), Kruskal–Wallis with Dunn’s post hoc test,cfrom left to right **p= 0.0017,p> 0.9999,p> 0.9999, Kruskal–Wallis with Dunn’s post hoc test,d*p= 0.0494 (WT),p> 0.9999 (Tlr2-/-), Kruskal–Wallis with Dunn’s post hoc test,e**p= 0.0014 (WT), **p= 0.0026 (Tlr2-/-), one-way ANOVA with Sidak’s post hoc test andp= 0.0162 (WT),p= 0.0400 (Tlr2-/-), Kruskal–Wallis with Dunn’s post hoc test,f*p= 0.0142 (WT),p= 0.9898 (Tlr2-/-), one-way ANOVA with Sidak’s post hoc test andp= 0.2056 (WT),p> 0.9999 (Tlr2-/-), Kruskal–Wallis with Dunn’s post hoc test. Source data are provided as a Source Data file. Cell isolations and stimulations Bone marrow neutrophils were isolated from the femurs of mice by Histopaque density gradient centrifugation [67] and purity was confirmed to be >80% Ly6G + neutrophils by flow cytometry. P. melaninogenica lipoproteins were prepared by Triton X-114 phase partitioning [68] and P. melaninogenica LPS was prepared using an LPS isolation kit (Sigma). Concentrations were determined relative to Pam3SK4 and E. coli LPS standard curves by running purified lipoprotein and LPS preparations on a 15% sodium dodecyl-sulfate polyacrylamide gel electrophoresis gel prior to detection using a Silver Stain Kit (Bio-Rad Laboratories, Inc) and imaging on a ChemiDoc XRS + Gel Imaging System (Bio-Rad Laboratories, Inc). P. melaninogenica LPS endotoxin activity was confirmed using a Pierce™ Chromogenic Endotoxin Quant Kit (ThermoFisher Scientific). Lipoprotein lipase-treated P. melaninogenica HK was prepared by incubation with 200 μg lipoprotein lipase (Sigma) for 2 h at 37 °C. For cell stimulation assays, 10 5 neutrophils in RP10 media supplemented with penicillin and streptomycin were exposed to P. melaninogenica HK (1:1 ratio), lipase-treated P. melaninogenica HK, P. melaninogenica lipoprotein (10 ng/mL), P. melaninogenica LPS (10 ng/mL), C29 TLR2 inhibitor (100–200 μM, Selleck Chemicals), Resatorvid TAK-242 TLR4 inhibitor (100–200 μM, Selleck Chemicals), or Pam3SK4 (10 ng/mL, InvivoGen, San Diego, CA) and incubated for 24 h at 37 °C with 5% CO 2 prior to supernatant collection. For cell infection assays, 10 5 neutrophils were exposed to 10 5 S. pneumoniae for 1 h prior to washing and incubation for 24 h at 37 °C with 5% CO 2 with or without P. melaninogenica HK (1:1 ratio) in media containing gentamycin (10 μg/mL). Neutrophil functional assays Lung neutrophils were isolated by positive selection (MojoSort PE-positive selection kit, BioLegend), and purity was confirmed to be >90% Ly6G + neutrophils by flow cytometry. Similar results were obtained using lung neutrophils isolated by negative isolation (19762, Mouse Neutrophil Enrichment kit, STEMCELL Technologies). Neutrophils were isolated from the lungs of mice following 24 h treatment with PBS, E. coli LPS, or P. melaninogenica HK i.t. as indicated. 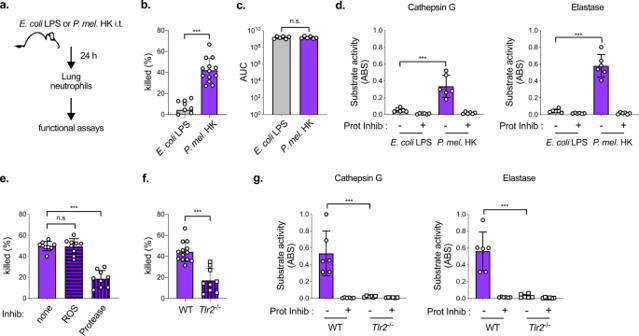Fig. 7:P. melaninogenica(P. mel.) enhances serine protease-mediated killing ofS. pneumoniaeby lung neutrophils in a TLR2-dependent manner. aSchematic of lung neutrophil purification.bPercent of type 2S. pneumoniaekilled by lung neutrophils purified from mice exposed to eitherE. colilipopolysaccharide (LPS) orP. mel. strain 25845 heat-killed (HK) i.t. for 24 h following 1 h incubation withS. pneumoniaeopsonized with 3% fresh mouse serum (n= cells isolated from 11 mice/group).cTotal reactive oxygen species (ROS) produced in 1 h by lung neutrophils purified from mice exposed to eitherE. coliLPS orP. mel. HK i.t. for 24 h detected by luminol, with area under curve (AUC) shown (n= cells isolated from 6 mice/group).dSerine protease activity for cathepsin G and elastase + /– protease inhibitor cocktail (Prot Inhib) detected by substrate cleavage for lung neutrophils purified from WT mice exposed to eitherE. coliLPS orP. mel. HK (n= cells isolated from 6 mice/group).ePercent ofS. pneumoniaekilled by lung neutrophils purified from WT mice exposed toP. mel. HK i.t. for 24 h following 1 h incubation with opsonizedS. pneumoniaein the presence of the ROS inhibitor DPI (ROS), protease inhibitors (Protease), or no inhibitors (none), (n= cells isolated from 9 mice/group).f,gPercent ofS. pneumoniaekilled by lung neutrophils purified from WT orTlr2-/-mice exposed toP. mel. HK i.t. for 24 h (n= cells isolated from 13 WT mice, 9Tlr2-/-mice) (f) or serine protease activity +/– protease inhibitor cocktail (Prot Inhib) (n= cells isolated from 6 mice/group) (g). Data are pooled from three independent experiments, with cells plated in duplicate or triplicate. Data are displayed as mean ± SEM. Forb***p< 0.0001, two-tailedt-test,cp= 0.9566, two-tailedt-test,d***p= 0.0004 (Cathepsin G), ***p< 0.0001 (Elastase), two-tailedt-test,ep= 0.9926 (ROS), ***p< 0.0001 (Protease), one-way ANOVA with Dunnett’s post hoc test,f***p< 0.0001, two-tailedt-test,g***p= 0.0008 (Cathepsin G), ***p= 0.0002 (Elastase), two-tailedt-test. Source data are provided as a Source Data file. For opsonophagocytic killing assays, 10 3 S. pneumoniae grown to mid-log phase were opsonized for 30 min with 3% fresh mouse sera prior to incubation with 10 5 neutrophils in Hank’s buffer/0.1% gelatin for 1 h at 37 °C under rotation. Killing assays were completed in the presence or absence of 1x Halt™ protease inhibitor cocktail (ThermoFisher Scientific) or 10 μM diphenyleneiodonium chloride (DPI), (ThermoFisher Scientific), which we found did not impact neutrophil viability over the course of 1 h. CFUs were measured by serial dilution plating, and percent killing was determined relative to reactions without neutrophils. Serine protease activity was determined using substrates specific to elastase (0.85 mM MeOSuc-Ala-Ala-Pro-Val- p NA, Sigma) and cathepsin G (0.1 mM Succinyl-Ala-Ala-Pro-Phe-pNA, Sigma) [58] . Briefly, 10 5 purified neutrophils were incubated with or without 1x Halt™ protease inhibitor cocktail for 30 min prior to washing and lysis in 0.1% Triton X-100. Substrates were added to neutrophil lysates and incubated in the dark for 45 min at 37 °C. Absorbance was determined by reading the OD 410 on Synergy™ HT Microplate Reader (BioTek) minus control wells with no neutrophils added. For detection of total ROS, 10 5 purified neutrophils were resuspended in KRP buffer (5 mM glucose, 1 mM CaCl 2 , 1 mM MgSO 4 in PBS) and equilibrated for 15 min prior to plating on Greiner Bio-One LUMITRAC™ plates (FisherScientific) followed by the addition of 50 μM luminol (FisherScientific) [69] . Luminescence over 1 h at 37 °C was detected using a Synergy™ HT Microplate Reader (BioTek). Area under curve (AUC) was calculated, minus wells with no neutrophils added. 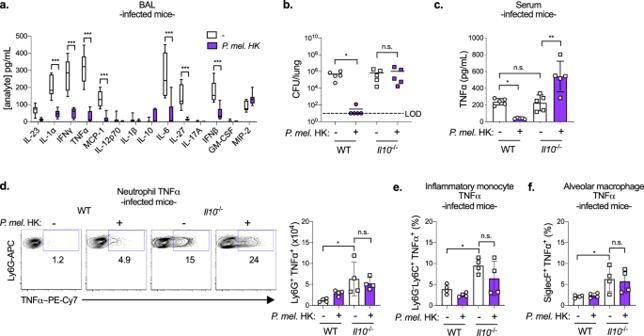Fig. 8:P. melaninogenica(P. mel.)-mediated protection againstS. pneumoniaerequires restraint of detrimental inflammation by IL-10. aQuantification of cytokines and chemokines in lung bronchoalveolar lavage (BAL) following exposure to PBS (-) orP. mel. strain 25845 heat-killed (HK) i.t. prior to 24 h type 2S. pneumoniaeinfection, 5 × 106CFU/mouse (n= 9 mice/group).b,cLungS. pneumoniaeburdens (b) and serum TNFα (c) detected in WT orIl10-/-mice exposed to either PBS (-) orP. mel. HK i.t. prior to 24 hS. pneumoniaeinfection (n= 5 mice/group).d–fRepresentative flow cytometry plots and total cell numbers of neutrophil TNFα (d), percentage of inflammatory monocyte TNFα (e), and percentage of AM TNFα (f) detected by intracellular flow cytometry from WT orIl10-/-mice treated with either PBS (-) orP. mel. HK i.t. prior to 24 hS. pneumoniaeinfection (n= 4 mice/group). LOD = limit of detection. Data are pooled from three independent experiments (a) or representative from one of four independent experiments (b–f). Box boundaries in (a) indicate the 25th and 75th percentiles, with a horizontal line representing the median and whiskers indicating minimum and maximum values. Data inb–fare displayed as mean ± SEM. Fora***p< 0.0001, two-way ANOVA with Sidak’s post hoc test,b*p= 0.0257 (WT),p> 0.9999 (Il10-/-), Kruskal–Wallis with Dunn’s post hoc test,cfrom left to right *p= 0.0393,p= 0.9973, **p= 0.0012, one-way ANOVA with Tukey’s post hoc test,dfrom left to right *p= 0.0116,p= 0.7388, one-way ANOVA with Sidak’s post hoc test (e), from left to right *p= 0.0101,p= 0.1698, one-way ANOVA with Sidak’s post hoc test,ffrom left to right *p= 0.0280,p= 0.9298, one-way ANOVA with Sidak’s post hoc test. Source data are provided as a Source Data file. 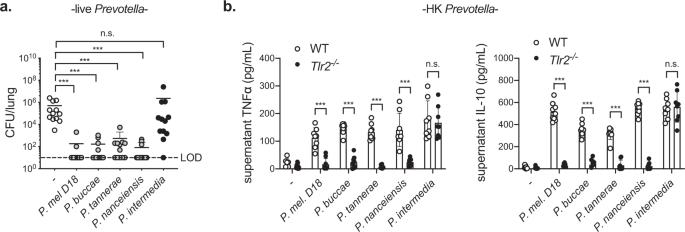Fig. 9: Protection againstS. pneumoniaeis induced by other airwayPrevotellathat activate neutrophils in a TLR2-dependent manner. aLungS. pneumoniaeburdens in mice treated with PBS (-), liveP. melaninogenica(P. mel.) strain D18, liveP. buccae, liveP. tannerae, liveP. nanceiensis, or liveP. intermediai.t. prior to 24 hS. pneumoniaeinfection, 5 × 106CFU/mouse (n= 12 mice/group).bSupernatant cytokines detected 24 h following incubation of BM neutrophils withP. mel. strain D18 heat-killed (HK),P. buccaeHK,P. tanneraeHK,P. nanceiensisHK, orP. intermediaHK (n= 3 independent experiments/group). Data are pooled from three independent experiments, with cells plated in triplicate for in vitro studies, displayed as mean ± SEM. Forafrom left to right ***p< 0.0001, ***p< 0.0001, ***p= 0.0005, ***p< 0.0001,p= 0.9999, Kruskal–Wallis with Dunn’s post hoc test,bfrom left to right, ***p< 0.0001, ***p< 0.0001, ***p< 0.0001, ***p< 0.0001,p= 0.9959 (TNFα), ***p< 0.0001, ***p< 0.0001, ***p< 0.0001, ***p< 0.0001,p= 0.9948 (IL-10), two-way ANOVA with Sidak’s post hoc test. Source data are provided as a Source Data file. Study approval These studies were approved by the Animal Care and Use Committee of the University of Colorado School of Medicine (protocol #00927) and by the Institutional Biosafety Committee (protocol #1418). Statistical analysis All measurements were taken from distinct samples, with exact sample sizes indicated in Figure legends. Prism (GraphPad, version 8) was used for all statistical analysis. All data were tested for normality using the Shapiro–Wilk test. For data with normal distributions, two-tailed Student’s t -tests, one-way or two-way ANOVA tests with Dunnett’s, Sidak’s, or Tukey’s post hoc analyses for multiple comparisons were used as specified. Two-tailed Mann–Whitney U -tests and Kruskal–Wallis tests with Dunn’s post hoc analysis for multiple comparisons were used for all data with non-Gaussian distributions. Log-rank Mantel-Cox test was used for survival group comparison. For all statistical tests, p -values < 0.05 was considered significant. Individual p -values are specified in Figure Legends. Reporting summary Further information on research design is available in the Nature Research Reporting Summary linked to this article.